SUMOylation of VEGFR2 regulates its intracellular trafficking and pathological angiogenesis Regulation of VEGFR2 represents an important mechanism for the control of angiogenesis. VEGFR2 activity can be regulated by post-translational modifications such as ubiquitination and acetylation. However, whether VEGFR2 can be regulated by SUMOylation has not been investigated. Here we show that endothelial-specific deletion of the SUMO endopeptidase SENP1 reduces pathological angiogenesis and tissue repair during hindlimb ischemia, and VEGF-induced angiogenesis in the cornea, retina, and ear. SENP1-deficient endothelial cells show increased SUMOylation of VEGFR2 and impaired VEGFR2 signalling. SUMOylation at lysine 1270 retains VEGFR2 in the Golgi and reduces its surface expression, attenuating VEGFR2-dependent signalling. Moreover, we find that SENP1 is downregulated and VEGFR2 hyper-SUMOylated in diabetic settings and that expression of a non-SUMOylated form of VEGFR2 rescues angiogenic defects in diabetic mice. These results show that VEGFR2 is regulated by deSUMOylation during pathological angiogenesis, and propose SENP1 as a potential therapeutic target for the treatment of diabetes-associated angiogenesis. Angiogenesis, the formation and maintenance of blood vessels architecture from pre-existing vessels, plays important roles in physiological as well as pathological settings such as ischemia, inflammation, diabetes, and cancer [1] . Vascular endothelial cell growth factors (VEGFs) and their cognate receptors (VEGFRs) have been identified to be critical in regulating vessel formation in angiogenesis [2] , [3] . VEGF primarily activates VEGFR2 (also known as Flk-1 or KDR)-mediated signaling cascadse to induce angiogenic responses; these signalling pathways include activation of phospholipase C-γ (PLC γ)–ERK1/2 pathway, PI3K–AKT–mTOR pathway, SRC kinases and small GTPases pathways that are involved in cell survival, cell migration and polarization, as well as regulation of endothelial junctions, vascular barrier function and vasomotion during vascular development. Given the critical role of VEGFR2 signalling in angiogenesis, regulation of VEGFR2 activity/activation may represent an important mechanism for the control of angiogenesis. The cell surface concentration of VEGFR2 dictates the level of VEGF signalling, with high concentrations lead to sustained signalling [4] , [5] . Endocytosis of VEGFR2 and regulation of VEGFR2 signalling has been extensively reported. Upon VEGF stimulation, activated/dimerized VEGFR2 undergo internalization via Ephrin-B2 and Par3-DAB2 complex [6] , [7] . Small GTPase ARF6 can mediate both internalization and recycling, which is regulated by two ARF6 guanine nucleotide exchange factors (GEFs) ARNO and GEP100, respectively [8] . VEGFR2 intracellular trafficking requires the synectin–myosin-VI complex, which is recruited by neuropilin-1 (NRP1) after receptor internalization [9] , [10] . At molecular levels, the PDZ binding motif on NRP1 mediates binding to the PDZ domain of synectin, which forms a complex with myosin-VI via its myosin-VI binding motif. Moreover, increased VEGFR2 intracellular trafficking could prevent activated VEGFR2 from inactivation by phosphatases [11] . Alternatively, it seems that a pool of VEGFR2 is ubiquitinated and their endocytosis is mediated by epsin, a family of ubiquitin binding endocytic clathrin adaptor protein, promoting endocytosis and degradation of VEGFR2 in EC [12] . Consistently, VEGFR2 could be negatively regulated by E3 ubiquitin ligase c-Cbl and SCF βTRCP -dependent ubiquitination and degradation [13] , [14] , [15] . However, whether or not VEGFR2 is regulated SUMOylation, a conjugation by ubiquitin-like small molecule (SUMO) on lysine residues, has not been investigated. SUMOylation is a post-translational modification that a target protein is covalently conjugated with the small ubiquitin-like modifier (SUMO) to specific lysine residues through formation of isopeptide bonds [16] , [17] . A consensus sequence ØKXE (Ø is a large hydrophobic amino acid and K is the site of SUMO conjugation) has been identified as the SUMO acceptor site [17] . SUMO modification regulates a variety of protein functions, including protein localisation, protein–protein interaction, protein–DNA interaction, and/or protein activity. However, the effect of SUMOylation on protein function is substrate specific. Protein SUMOylation is dynamically regulated by activating (E1), conjugating (E2), and ligating (E3) enzymes, but can be reversed by a family of SUMO-specific proteases (SENPs) [18] , [19] . Six SENPs have been identified, and they have distinct expression profiles, substrate specificities and cellular localisation [18] . SENP1 and SENP2 have broad specificity for the three mammalian SUMOs (SUMO1–3), while SENP3, SENP5, SENP6, and SENP7 prefer SUMO2/3 as substrates. SENP1 is a protease that appears to be localised in several compartments and deconjugates a great number of SUMOylated proteins [18] . We and others have reported that a global deletion of SENP1 gene in mice causes perinatal lethality due to defects in erythropoiesis [20] , [21] . We also observed delayed vascular formation in SENP1 global knockout mice [20] . The role of SENP1 in endothelial cells and angiogenesis has been examined. Specifically, it is reported that induction of SENP1 in endothelial cells contributes to hypoxia-derived VEGF expression and angiogenesis in vitro [22] . We have recently reported that endothelial SENP1 also suppresses Notch overactivation and contributes to normal retinal sprouting at neonatal stages [23] . However, the role of SENP1 in pathological angiogenesis has not been investigated. In the present study, we show that SENP1 is highly expressed in vascular endothelial cells (EC) in response to ischemia. Mice with an EC-specific deletion of SENP1 (SENP1-ECKO) exhibit reduced ischemia-induced and VEGF-induced pathological angiogenesis. Mechanistic studies indicate that VEGFR2 is SUMOylated and accumulated at the Golgi in the absence of SENP1, attenuating VEGFR2 surface expression and signalling. Therefore, our data suggest that SENP1 keeps VEGFR2 in a deSUMOylated state to ensure VEGFR2 membrane targeting in EC, uncovering a novel mechanism for VEGFR2 regulation. SENP1 deletion attenuates pathological angiogenesis We observed a delayed vascular formation in the SENP1 global knockout mice, which suggested that SENP1 might be involved in regulation of angiogenesis [20] . We further explored this possibility in mice with vascular EC-specific deletion of SENP1 (SENP1-ECKO), which was generated by mating SENP1 lox/lox with VE-cadherin-Cre mice followed by breeding to C57BL/6 background [24] , [25] (Supplementary Fig. 1a ). Real-time RT-PCR and immunofluorescence staining revealed an efficient endothelial deletion of SENP1 in CD31 + NG2 − mouse brain microvascular EC (MBMVEC) [26] , but not in CD31 − NG2 + mouse brain microvessel pericytes (MBMVPC) isolated from SENP1-ECKO mice (Supplementary Fig. 1b-c ). Retina sprouting in neonatal SENP1-ECKO is delayed due to increased Notch signalling [23] , but was similar to WT mice after day 9 (Supplementary Fig. 2 ). SENP1-ECKO did not exhibit obvious vascular defects with normal breeding and growth compared to SENP1 lox/lox or normal C57BL/6 mice in adulthood (see next sections for hindlimb, ear skin, and retina). To investigate if SENP1 gene is critical for adaptive angiogenesis, SENP1 lox/lox (WT) and SENP1-ECKO mice were subjected to femoral artery ligation by surgical arterectomy of the left femoral artery as we reported recently [27] - [29] . In this model, a decreased number of capillaries surrounding each muscle fiber (capillary/fiber ratio) results in a decrease in calf blood pressure ratios and blood flow, leading to incapability to mount an adaptive angiogenic response [28] . Blood flow in both ischemic and non-ischemic limb perfusion pre-surgery and post-surgery at indicated timeframe (3 days, 1 week, 2 weeks, and 4 weeks) were measured, and the ratio of left leg to right leg gastrocnemius blood flow was set as 1 before surgery. This ratio in WT mice dropped by 80% immediately after the surgery but gradually recovered over 4 weeks. However, an attenuated recovery of hindlimb perfusion and flow were observed in SENP1-ECKO mice (Fig. 1a ). A decreased arteriogenesis from existing vessels of the upper limb and decreased neovascularization/vessel maturation in the lower limb could contribute to impaired limb perfusion [28] , [29] . Ischemia-induced arteriogenesis measured by microfil casting followed by 3D Micro-CT [11] was greatly reduced in SENP1-ECKO mice (Fig. 1b with quantifications in 1c, d). Angiogenesis and vessel maturation in gastrocnemius muscles measured by immunostaining with anti-CD31 and smooth muscle actin were also impaired in SENP1-ECKO mice (Fig. 1e with quantification of capillary number/mm 2 and ratio of capillary/fiber in Fig. 1f, g ). Fig. 1 SENP1-ECKO mice exhibit attenuated arteriogenesis and angiogenesis in vivo. WT and SENP1-ECKO mice were subjected to hindlimb ischemic ligation model (HLI). a Laser Doppler analysis of blood flow. The graph shows blood flow in the ischemic foot expressed as a ratio to flow in the normal foot. Quantitative analysis of laser Doppler images indicates significant alterations in hindlimb reperfusion starting at 7 days after femoral artery ligation in SENP1-ECKO mice relative to WT mice ( n = 6 each strain). b Representative micro-CT images of WT and SENP1-ECKO mice 14 days after HLI. c , d Quantitative micro-CT analysis of arterial vasculature above and below the knee in WT mice ( n = 6500 cross-sections per mouse) and SENP1-ECKO mice ( n = 4500 cross-sections per mouse) 14 days after common femoral artery ligation. Note a marked decrease in total number of <120-μm-diameter vessels in SENP1-ECKO mice relative to WT littermates in thigh and calf (mean ± SEM, * P < 0.05). Statistical significance was assessed using a Mann–Whitney U test and repeated measures analysis performed using one-way nonparametric ANOVA (Kruskal Wallis test). e – g Attenuated angiogenesis in SENP1-ECKO mice. Capillary density was immunostained with an EC marker CD31. Representative sections from non-ischemic and ischemic groups of WT and SENP1-ECKO mice on day 28 post-ischemia are shown in ( e ). Quantification of capillary density (number/mm 2 muscle area) and ratio of CD31/myocyte are shown in ( f , g ). Data are mean ± SEM from ten fields per section (three sections/mouse and n = 4 for each strain). h – j Attenuated VEGF-VEGFR2 signalling in SENP1-ECKO. Muscle tissues from WT and SENP1-ECKO were harvested at various days post-ischemia as indicated. h HIF-1α, SENP1, and β-actin were determined by western blot with respective antibodies. i VEGF-A mRNA was measured by qRT-PCR with GAPDH for normalization. Fold changes are presented. n = 2 per group. j Phosphorylations of VEGFR2, Akt, and ASK1 as well as total proteins as indicated in tissue lysates were determined by western blot with respective antibodies. SUMOylated VEGFR2 was determined by co-immunoprecipitation assays with anti-SUMO1 followed by western blotting with anti-VEGFR2. Protein bands in ( h , j ) were quantified by densitometry and fold changes are presented by taking WT non-ischemia as 1.0. n = 2. Error bars, mean ± SEM; ∗ P < 0.05, ** P < 0.01, one-way ANOVA. Scale bar: 500 μm ( b ); 20 μm ( e ) Full size image The hindlimb ischemia model represents pathological settings involving inflammation, multiple cytokines, and proangiogenic factors [27] . SENP1 has been shown to stabilize HIF1α and HIF1α-dependent VEGF transcription [21] . Indeed, we observed a decrease in HIF1α protein and VEGF-A mRNA under hypoxia in SENP1 knockdown ECs compared to WT ECs (Supplementary Fig. 3a, b ). We examined SENP1 and HIF1α protein as well as VEGF mRNA levels in the ischemic hindlimb tissues of WT and SENP1-ECKO. SENP1 protein was upregulated in WT mice in response to ischemia and only weakly detected in the SENP1-ECKO muscle tissues (Fig. 1h ), suggesting that the SENP1 protein was induced by ischemia primarily in the vascular endothelium. This was further confirmed for SENP1 expression in ischemic hindlimb by immunohistochemistry (Supplementary Fig. 3c ). Despite that HIF1α protein was markedly decreased at day 3 post-ischemia in SENP1-ECKO mice, we did not observe significant differences between the two groups in VEGF mRNA levels (Fig. 1h, i ). This suggest that other cell types such as myocyte rather than EC primarily contributes to VEGF-A expression in ischemic hindlimb. SENP1-mediated ASK1 activation (p-ASK1), which is known to mediate inflammation and cellular apoptosis [30] , [31] , was not significantly attenuated by SENP1 deletion in ischemic muscle. These data suggest that ASK1 signaling did not contribute to reduced macrophage infiltration (Supplementary Fig. 3d-e ) and cell death (TUNEL assay) in ischemic hindlimb of SENP1-ECKO (Supplementary Fig. 3f-g ). We have previously shown that VEGFR2 signalling plays critical roles in ischemia-mediated arteriogenesis and angiogenesis [28] , [29] . An extra band of VEGFR2 with molecular shift was detected in the SENP1-ECKO hindlimb tissues, and was verified as SUMOylated VEGFR2 by co-immunoprecipitation assays with anti-SUMO1 followed by western blotting with anti-VEGFR2. Phosphorylation of VEGFR2 and its downstream phosphor-Akt were induced in response to ischemia in WT mice. These responses were drastically reduced in the SENP1-ECKO hindlimb (Fig. 1j ). These data suggest that endothelial deletion of SENP1 attenuates VEGFR2 signalling and pathological angiogenesis in mouse models. SENP1 deletion impairs VEGF-induced neovascularization As the role of SENP1 in regulation of VEGFR2 has not been explored, we therefore focused on SENP1-VEGFR2 in our subsequent studies. To directly determine the role of SENP1 in regulating VEGFR2-dependent angiogenesis in vivo, we performed VEGF-induced tissue angiogenesis assays in SENP1-ECKO mice. Adenovirus encoding VEGF-A 164 (Ad-VEGF) or β-gal was injected into ear intradermally or into the eye intravitreously for ear angiogenesis and retinal angiogenesis, respectively. VEGF-induced angiogenesis was accessed by a whole-mount CD31 or isolectin staining (Fig. 2a, b, c for ear and Fig. 2d, e, f for retina). We also examined angiogenesis in the avascular cornea into which recombinant VEGF protein formulated into Hydron pellets was implanted (Fig. 2g, h, i ). In all these assays, VEGF-induced angiogenesis was dramatically attenuated in SENP1-ECKO mice. These data suggest that SENP1 is critical for VEGFR2 activity and VEGF-induced angiogenesis. Fig. 2 VEGF-induced retina and cornea neovascularization were greatly attenuated in SENP1-ECKO mice. a – c VEGF-induced ear angiogenesis. Adenovirus encoding VEGF 164 (1 × 10 9 pfu) (Ad-VEGF) or β-galactosidase (Ad-LacZ) was intradermally injected into the mice right and left ear skin, respectively. a VEGF-induced angiogenesis in WT and SENP1-ECKO mice was accessed by a direct microscopy. b Ear vasculature was visualized by a whole-mount staining with PE-conjugated anti-CD31. c Quantification of vessel density from 10 fields per ear ( n = 5 for each group). d – f VEGF-induced retina angiogenesis. Ad-VEGF or Ad-LacZ (1 × 10 9 pfu) was injected intravitreously into WT and SENP1-ECKO mice. Retina vasculature was visualized by isolectin staining (low power images in ( d ) and high power images in ( e ) with quantification of vessel density in ( f ). g – i VEGF-induced cornea angiogenesis assay. A Hydron pellet containing VEGF protein was implanted into the cornea of WT and SENP1-ECKO mice. Angiogenesis was assessed by stereomicroscopy on day 5 following implantation ( g ) and immunostaining with anti-CD31 ( h ). Vascular density was quantified in ( i ). Quantificaitons were from ten fields per tissue (ear, retina or cornea) ( n = 5 for each group). Error bars, mean ± SEM; ∗ P < 0.05, ** P < 0.01, one-way ANOVA. Scale bar: 100 μm ( b , e , h ); 400 μm ( d ) Full size image SENP1-deficient EC attenuates VEGFR2 angiogenic signaling We then directly examined if SENP1 mediates VEGF-VEGFR2 angiogenic signalling by in vitro models for EC migration and tube formation. Silencing of SENP1 by siRNA in primary human EC (HUVEC) significantly blunted VEGF-induced EC migration in a monolayer “wound injury” assay (Fig. 3a, b ). The effects of SENP1 on EC cord formation were also determined in a Matrigel tube formation assay. Silencing of SENP1 in HUVEC significantly attenuated VEGF-induced EC tube formation as quantified for the number of cords and branches (Fig. 3c, d ). We also performed a 3D spheroid sprouting assay in which ECs were coated onto cytodex beads following by embedding in fibrin gels. Fibroblasts cultured on top of the gel promoted optimal sprouting and tube formation which peaked at day 8 [26] . Quantitative analyses indicated that the number of sprouts was drastically reduced by SENP1 depletion (Fig. 3e, f ). In line with our recent study [32] , we observed a significant reduction of GATA2 in siSENP1 transfected EC. While SENP1 knockdown by siRNA had no effects on VE-cadherin, VEGF-induced phosphor-VEGFR2 and its downstream Akt were reduced by SENP1 siRNAs in HUVEC (Fig. 3g, h ). We observed similar effects of SENP1 deficiency on VEGF-induced EC migration and VEGFR2 signalling in isolated mouse brain microvessel ECs (MBMVECs). Moreover, re-expression of SENP1 rescued the defects in VEGF-VEGFR2 angiogenic signalling caused by SENP1 deficiency in MBMVEC (Supplementary Fig. 4 ). Taken together, these in vivo and in vitro results support a critical role of SENP1 in mediating VEGFR2 angiogenic signalling. Fig. 3 VEGF-induced angiogenic responses were inhibited by SENP1 silencing. HUVEC were transfected with control siRNA (siCtrl) or SENP1 siRNA (siSENP1) for 24 h. Cells were cultured in 0.5% FBS for overnight and subjected to EC migration and tube formation in response to VEGF (10 ng/ml). a , b EC migration by a scratch assay for indicated times. Wound healing (% closure) was quantified. c , d EC tube formation in a Matrigel assay. Representative images are shown in ( c ). Number of cords and branches were quantified from ten fields per group ( d ). e , f 3D spheroid sprouting assay. siRNA-transfected HUVECs were infected with EGFP-expressing retroviruses. Cells were coated with microbeads, embedded in fibrin gels and grown in EGM2 medium for 8 days. e A representative image of ten beads for each sample is shown. f Quantification of sprout number is shown in panel. Three independent experiments were performed. g , h Ctrl siRNA and SENP1 siRNA HUVEC were cultured overnight in 0.5% FBS followed by VEGF treatment (10 ng/ml) for indicated times (0–15 min). g Phosphorylation of VEGFR2 and Akt as well as the total proteins as indicated were determined by western blot with respective antibodies. h Protein bands were quantified by densitometry and fold changes are presented by taking untreated siCtrl group as 1.0. n = 2. Error bars, mean ± SEM; ∗ P < 0.05, Student t -test ( f ) or one-way ANOVA. Scale bar: 1 mm ( a , c , e ) Full size image VEGFR2 SUMOylation retains VEGFR2 in the Golgi Given that the total VEGFR2 was not affected in SENP1-deficeint ECs, we examined if the intracellular localisation of VEGFR2 was altered by the SENP1 deficiency to attenuate VEGFR2 signalling. Immunofluorescence staining indicated that VEGFR2 was primarily detected on EC surface of normal MBMVEC. However, SENP1 deficiency induced a profound accumulation of VEGFR2 at the Golgi where it was co-localised with GM130 (Fig. 4a ). In contrast, the surface localisation of TNF-receptor 2 (TNFR2) was not affected by the SENP1 deletion (Fig. 4b ). Similar effects of SENP1 deletion on VEGFR2 and TNFR2 were obtained in HUVEC by siRNA silencing (Supplementary Fig. 5a ). The kinesin family plus-end molecular motor KIF13B has been shown to deliver VEGFR2 from the Golgi to the EC surface [33] . Indeed, knockdown of KIF13B in HUVEC caused VEGFR2 accumulation at the Golgi (Supplementary Fig. 5b ). Furthermore, the reduced surface expression of VEGFR2 in SENP1-deficient ECs was confirmed by a cell-surface biotinylation assay (Fig. 4c ) [12] . Accordingly, SUMOylated VEGFR2 was augmented in SENP1-ECKO MBMVEC as detected by a co-immunoprecipitation assay (Fig. 4d ). To determine a physiological relevance of VEGFR2 SUMOylation, we examined if VEGFR2 SUMOylation and Golgi accumulation were agonist dependent. We observed that VEGF-induced VEGFR2 SUMOylation concomitant with its Golgi localisation, peaking at 15 min upon VEGF-engagement (Fig. 4e, f ). Fig. 4 SUMOylation of VEGFR2 at the C-terminal lysine-1270 retains VEGFR2 in the Golgi. a , b . MBMVEC isolated from WT and SENP1-ECKO mice were subjected to immunofluorescence staining for VEGFR2 ( a ) or TNFR2 ( b ) together with a Golgi marker GM130. c WT and SENP1-ECKO MBMVECs were cultured in normal media. Cell-surface VEGFR2 was labeled by cell-surface biotinylation, and analyzed by streptavidin bead pull-down followed by western blotting with anti-VEGFR2. Percentage of cell-surface vs total proteins (VEGFR2, TNFR2 and actin) were quantified. n = 2. d Cell lysates of MBMVEC isolated from WT and SENP1-ECKO mice were subjected to western blot for total SENP1, VEGFR2, and co-immunoprecipitation assays for VEGFR2 SUMOylation. Relative molecular weights are shown on the left. e WT MBMVEC were treated with VEGF (10 ng/ml) for indicated times, and cells were subjected to immunofluorescence staining for co-localisation of VEGFR2 with GM130 ( e ). f Schematic diagram of VEGFR2 domains. EM: extracellular domain, TM: transmembrane domain, IM: intracellular domain, Tail: a flexible C-terminal segment (residues aa1172–1356). The numbers refer to the amino acid number, indicating the boundary of each domain. Y1054/59 located at the activation loop and putative SUMO sites within the IM (K1110, K1120, and K1270) are indicated. All VEGFR2 expression constructs are Flag-tagged at the N termini. g VEGFR2-WT and mutants were transfected into WT or SENP1-deficient MBMVEC. Co-localisation of VEGFR2 (anti-FLAG) with GM130 was determined. Merged images are shown (see Supplementary Fig. 6 for split channel images). A total of 10 cells from each group were analyzed. Golgi-accumulated VEGFR2 is indicated by arrows while membrane/cytosolic VEGFR2 by asterisks ( a , b , e , g ). TNFR2 was absent in Golgi ( b ). Three independent experiments were performed. Scale bar, 20 μm ( a , b , e , g ) Full size image SENP1 is an endopeptidase that deconjugates SUMOs off substrate proteins. Our data indicated that VEGFR2 was SUMOylated in SENP1-deficient tissues and ECs. We reasoned that SUMOylation-modified VEGFR2 was accumulated at the Golgi. To test this hypothesis, bioinformatics analyses for the amino acid sequence of VEGFR2 protein indicated that VEGFR2 contains several putative SUMOylation sites (Lys1110, Lys1120 and Lys1270) at the C-terminal domain (Fig. 4f ), K286 located at the extracellular domain and K729 at the kinase domain (not depicted in the figure). We first generated VEGFR2 truncated mutants with a deletion of the C-terminal domain (VEGFR2-ΔC) or the kinase domain (VEGFR2-ΔK) (Supplementary Fig. 6a ). VEGFR2-WT, when was expressed in HUVECs, could be detected at the Golgi. VEGFR2-ΔC, but not VEGFR2-ΔK, abolished the Golgi localisation (Supplementary Fig. 6b ). We then generated mutant VEGFR2 bearing Lys (K) to Arg (R) substitution at a single residue (K1110R, K1120R, and K1270R) or at all three residues (triple KR; TKR) by site-specific mutagenesis. Mutant VEGFR2 was expressed in both normal and SENP1-deficient MBMVECs to determine its cellular localisation. VEGFR2-WT was distributed on plasma membrane in normal ECs. However, SENP1 deletion induced a Golgi accumulation. Interesting, the mutation at K1270 (K1270R or TKR) diminished the accumulation of VEGFR2 at the Golgi in ECs (Fig. 4g ; Supplementary Fig. 6c-d for split channel images). These results suggest that a potential modification of VEGFR2 at K1270 induces its Golgi accumulation in SENP1-deficient ECs. SUMOylation inhibits VEGFR2-mediated angiogenesis To directly determine how SUMOylation regulates VEGFR2 activity and angiogenic signalling, we generated a construct expressing VEGFR2-SUMO1 fusion protein, a well-accepted approach in studying the function of SUMOylated proteins [16] , [20] . Since K1270 is proximal to the C-terminus of VEGFR2, VEGFR2-SUMO1 fusion with SUMO1 fusion to the VEGFR2 C-terminus would mimic the endogenous SUMOylated VEGFR2 (Fig. 5a ). While VEGFR2 was detected throughout the cells, VEGFR2-SUMO1 was completely accumulated at the Golgi (Fig. 5b ). To determine if the aberrant compartmentalization of VEGFR2 reduces VEGFR2 activity and angiogenic signalling, we first examined effects of SUMO1 conjugation on VEGFR2 activity. VEGFR2-WT, VEGFR2 K1270R (a form that cannot be SUMOylated) or VEGFR2-SUMO1 (a form that is constitutively SUMOylated) was expressed in HUVEC by lentivirus infection, and VEGF-induced p-VEGFR2 was examined by western blotting. Compared to the vector control, VEGFR2 expression in HUVEC induced autophosphorylaton of VEGFR2-WT. While VEGFR2 K1270R showed slightly stronger than WT in VEGF-induced VEGFR2 tyrosine phosphorylation, SUMO1 fusion to VEGFR2 diminished its autophoshorylation (Fig. 5c, d ). Function of VEGFR2 SUMOylation on EC migration in a monolayer “wound injury” assay was determined by expressing VEGFR2-WT, VEGFR2-SUMO1 or VEGFR2-K1270R mutant into HUVEC. Expression of VEGFR2-WT or VEGFR2-KR augmented VEGF-induced EC migration compared to the vector control cells. However, VEGFR2-SUMO1 significantly blunted VEGF-induced EC migration (Fig. 5e, f ). We then examined the effects of VEGFR2 SUMOylation on in vivo angiogenesis in the mouse models. To this end, adenovirus expressing VEGFR2-WT, VEGFR2-SUMO1 or VEGFR2-K1270R mutant was administrated into mice intravitreously. Adenoviral infection efficiency was determined by immunostaining with anti-FLAG for exogenously expressed VEGFR2 (Supplementary Fig. 7 ). VEGFR2-mediated angiogenesis was accessed by a whole-mount staining with isolectin staining. VEGFR2-WT or K1270R significantly augmented retinal sprouting, with VEGFR2-K1270R had more profound effects. In contrast, VEGFR2-SUMO1 potently attenuated retinal vascular angiogenesis (Fig. 5g with quantifications in 5 h). Taken together, these data support that SUMOylation of VEGFR2 attenuates VEGFR2 activity and its dependent angiogenic signalling. Fig. 5 SUMOylation of VEGFR2 blocks VEGFR2 surface targeting and VEGFR2-mediated angiogenesis. a Schematic diagram of VEGFR2-SUMO1 fusion compared to endogenous SUMOylated VEGFR2. b HUVECs were transfected with VEGFR2-WT or VEGFR2-SUMO1, and cells were co-immunostained with anti-VEGFR2 and GM130. Merged images with DAPI counterstaining (blue) are shown. A total of 10 cells from each group were analyzed. Golgi-accumulated VEGFR2 is indicated by arrows while membrane/cytosolic VEGFR2 by asterisks. c , d HUVECs were infected with lentivirus expressing empty vector (EV), VEGFR2-WT, VEGFR2-KR or VEGFR2-SUMO1 followed by VEGF treatment as indicated. Phosphor- and total VEGFR2 were examined by western blotting. Protein bands were quantified by densitometry and fold changes are presented by taking untreated VEGFR2-WT group as 1.0. n = 2. e , f HUVEC were infected with lentivirus expressing empty vector, VEGFR2-WT, VEGFR2-SUMO1 and VEGFR2-K1270R for 24 h. Cells were cultured in 0.5% FBS for overnight and subjected to EC migration in response to VEGF (10 ng/ml). Representative images are presented in ( e ) and wound healing (% closure) at 9 h was quantified in ( f ). Data are mean ± SEM from ten fields per group. Three independent experiments were performed. g , h VEGFR2-SUMO1 blunts retina angiogenesis. Ad-VEGF or Ad-LacZ (1 × 10 9 pfu) was co-injected intravetrously with VEGFR2-WT, VEGFR2-SUMO1 or VEGFR2-K1270R into 4 day-old pups. Retina was harvested on day 5 post-injection and retina vasculature was visualized by isolectin staining with confocal images in ( g ) with quantification of vessel density in ( h ). n = 5 for each group. Error bars, mean ± SEM; ∗ P < 0.05, one-way ANOVA. Scale bar, 20 μm ( b ); 1 mm ( e ); 100 μm ( g ) Full size image VEGFR2-SUMO1 knockin blunts EC angiogenesis To further determine if SUMOylation modulates VEGFR2 cell surface distribution and cellular function, we established endothelial cells expressing an endogenous VEGFR2-SUMO fusion protein using Clustered regularly interspaced short palindromic repeats (CRISPR)/CRISPR-associated protein 9 nuclease (Cas9)-mediated gene editing. Specifically, we designed a specific single-guide RNA (sgRNA) targeting the vicinity of the stop codon of KDR gene encoding VEGFR2 and a repair template containing targeting arms with exon 30 as 5′ arm and the 3′UTR of the KDR gene as 3′ arm flanking the SUMO1 cDNA. Upon CRISPR/Cas9-mediated DNA double-strand breaks were repaired through homologous-directed repair [34] , the SUMO1 cDNA was integrated into the KDR locus just before the termination signal in endothelial colony forming cell-derived ECs so that engineered KDR-SUMO1 EC expresses VEGFR2-SUMO1 fusion protein (Fig. 6a ; Supplementary Fig. 8 ). We examined cellular localisation and angiogenic activity of VEGFR2-SUMO1 fusion protein in engineered ECs. As observed for overexpressed VEGFR2-SUMO1, endogenous VEGFR2-SUMO1 in KDR-SUMO1 ECs was also exhibited a Golgi accumulation (Fig. 6b ) with reduced surface expression as confirmed by a cell-surface biotinylation assay (Fig. 6c ). Accordingly, VEGF-induced autophosphorylaton of VEGFR2-SUMO1 was abrogated (Fig. 6d, e ). For functional analyses, we performed a 3D spheroid sprouting assay using normal (WT) and KDR-SUMO1 knockin human EC. Quantitative analyses indicated that the number of sprout formation by KDR-SUMO1 ECs was drastically reduced compared to normal ECs (Fig. 6f, g ). Taken together, our results indicate that SUMOlation of VEGFR2 hinders VEGFR2 cell surface distribution and its angiogenic signalling. Fig. 6 VEGFR2-SUMO1 fusion in human EC inhibits VEGF-mediated angiogenesis. a Schematic diagram of KDR-SUMO1 knockin in human EC by CRISPR/Cas9-mediated gene editing. A specific sgRNA targeting the vicinity of the stop codon of KDR gene encoding VEGFR2 and a repair template containing targeting arms with exon 30 as 5′ arm and the 3′UTR of the KDR gene as 3′ arm flanking the SUMO1 cDNA. Upon CRISPR/Cas9-mediated DNA double-strand breaks were repaired through homologous-directed repair, the SUMO1 cDNA was integrated into the KDR locus just before the termination signal. The PCR primers used for screening for KDR-SUMO1 fusion clones are indicated. b WT human EC and KDR-SUMO1 knockin EC were subjected to immunofluorescence staining for co-localisation of VEGFR2 with GM130. Similar pattern localisation was observed in cells derived from additional two clones. c WT human EC and KDR-SUMO1 knockin EC were cultured in normal media. Cell-surface VEGFR2 was labeled by cell-surface biotinylation, and analyzed by streptavidin bead pull-down followed by western blotting with anti-VEGFR2. Percentage of cell-surface VEGFR2 vs total VEGFR2 in WT EC and KDR-SUMO1 EC were quantified. n = 3. d , e WT human EC and KDR-SUMO1 knockin EC were treated with VEGF (10 ng/ml) for indicated times, and cells were subjected to western blot for VEGFR2 phosphorylation ( c ). Protein bands were quantified by densitometry and fold changes are presented by taking untreated WT group as 1.0 ( d ). n = 2. f , g 3D spheroid sprouting assay. Human ECs were infected with EGFP-expressing retroviruses. Cells were coated with microbeads, embedded in fibrin gels and grown in EGM2 medium for 8 days. A representative image of ten beads for each sample is shown ( f ). Quantification of sprout number is shown in panel ( g ). Three independent experiments were performed. Error bars, mean ± SEM; * P < 0.05, one-way ANOVA. Scale bar: 20 μm ( b ); 1 mm ( f ) Full size image Pathological role of the SENP1-VEGFR2 angiogenic signaling Finally, we examined the pathological relevance of SENP1/VEGFR2-mediated angiogenesis. It is well known that diabetic conditions impair angiogenesis such as wound healing although the underlying mechanism is not fully understood [35] . It has been reported that hyperglycemia promotes ligand-independent phosphorylation of VEGFR2, and this VEGFR2 signalling occurs within the Golgi compartment and results in progressively decreased availability of VEGFR2 at the cell surface [36] , [37] . Based on these observations, we reasoned that SENP1-VEGFR2 angiogenic signalling could be impaired in diabetic settings. To this end, we first examined hyperglycemia could induce SENP1 downregulation and VEGFR2 accumulation at the Golgi. ECs were cultured under 5 mM or 25 mM glucose (hyperglycemia) for 72 h, and SENP1 expression, VEGFR2 SUMOylation and VEGFR2 localisation were determined. SENP1 expression was drastically downregulated concomitant with increased VEGFR2 SUMOylation (Fig. 7a ). VEGFR2 was accumulated at the Golgi under 25 mM glucose where it was co-localised with Golgi marker (Fig. 7b ). We then examined if this was the case at diabetic settings. To this end, we use streptozotocin (STZ)-induced type I diabetic mouse model (T1DM) which was verified by blood glucose levels (Supplementary Fig. 9 ). Although SENP1 expression was increased in whole brain lysates, it was significantly reduced in the vascular layers of retina and ear skin from STZ mice compared to normal groups (Fig. 7c ), suggesting that hyperglycemia effects on SENP1 expression is more profound in the vasculature. Indeed, SENP1 expression was drastically reduced in brain EC isolated from STZ mice compared to normal group (Fig. 7d ). Accordingly, VEGFR2 was accumulated at the Golgi of brain vascular EC isolated from T1DM mice (Fig. 7e ). We then use the STZ mice to determine VEGFR2-mediated angiogenesis in an adenovirus-expressing VEGF-induced ear angiogenesis model. Consistent with previous reports, STZ mice exhibited reduced VEGF-induced angiogenesis. However, co-expression of VEGFR2-WT or VEGFR2-KR, but not VEGFR2-SUMO1, could rescue the angiogenesis defects in STZ-induced diabetic mice. Again, VEGFR2-K1270R had more profound effects than VEGFR2-WT (Fig. 7f with quantifications in 7g, h). These results support a critical function of the SENP1-VEGFR2 angiogenic pathway in diabetes. Fig. 7 The SENP1-VEGFR2 signalling in diabetic angiogenesis. a , b HUVEC were cultured under 5 mM or 25 mM glucose for 72 h. Expression of SENP1 and VEGFR2 SUMOylation were determined ( a ). VEGFR2 localisation was determined by indirect immunofluorescence for VEGFR2 and GM130 ( b ). c Tissues from WT and STZ mice were harvested. SENP1 expression in brain (whole lysates), retina and ear skin (the vascular layer) was determined by western blot with anti-SENP1. d SENP1 expression in MBMVEC isolated from WT and STZ mice. Protein bands in ( c , d ) were quantified by densitometry and fold changes are presented by taking WT group as 1.0. n = 2. e VEGFR2 localisation in MBMVEC isolated from WT and STZ mice was determined by indirect immunofluorescence for VEGFR2 and GM130. f – h Adenovirus encoding VEGF 164 (1 × 10 9 pfu) (Ad-VEGF) or β-galactosidase (Ad-LacZ) was co-injected with empty vector, VEGFR2-WT, VEGFR2-SUMO1 or VEGFR2-K1270R intradermally into ear skin of SENP1-ECKO mice. VEGF-induced angiogenesis in WT and SENP1-ECKO mice was accessed by a whole-mount staining with anti-CD31 antibody. Vascular density was quantified and data are mean ± SEM from ten fields per mouse ear. ( n = 5 for each group). Error bars, mean ± SEM; * P < 0.05, one-way ANOVA. Scale bar: 20 μm ( b ); 100 μm ( f ) Full size image The perinatal lethality resulted from a SENP1 global deletion excluded further studies on the role of SENP1 in pathological angiogenesis. In the present study, we investigate the role of SENP1 in reparative angiogenesis using an EC-specific deletion of SENP1 (SENP1-ECKO). Our data demonstrate that SENP1-ECKO mice exhibit severe ischemia and VEGF-mediated angiogenesis. This is evident in a femoral artery ligation-induced ischemia hindlimb model and in VEGF-induced ear, retina, and cornea angiogenesis assays. We further demonstrate that SENP1 deletion in EC attenuates VEGF-induced VEGFR2 activation and VEGFR2-mediated angiogenesis in EC migration and tube formation assays. VEGFR2 could be modified by SUMOylation at Lys1270 which is drastically augmented in the absence of SENP1; this modification induces VEGFR2 accumulation at the Golgi, blocking VEGFR2 trafficking to cell surface and signalling. A specific mutation of Lys to Arg at 1270 abolishes the Golgi accumulation of VEGFR2, even in the SENP1-deficient EC. By using VEGFR2-SUMO1 fusion knockin mimicking the endogenous SUMOylated VEGFR2, we show that VEGFR2-SUMO1 significantly blunts VEGF-induced VEGFR2 signalling and angiogenic responses in EC. Expression of a SUMOylation-defective mutant VEGFR2-K1270R, but not SUMOylated form of VEGFR2 (VEGFR2-SUMO1), stimulates angiogenesis in vitro and in vivo. Moreover, we show that the SENP1-VEGFR2 signalling is impaired under hyperglycemia in vitro and at diabetic settings in vivo; the reduction of the SENP1-VEGFR2 signalling account for the impaired angiogenesis in diabetes as overexpression of non-SUMOylated form of VEGFR2 could rescue the angiogenic defects in STZ mice. Detailed mechanistic analyses support that SENP1 maintains VEGFR2 in an un-SUMOylated state, ensuring normal VEGFR2 trafficking and signalling in EC; pathological conditions such as hyperglycemia downregulate SENP1, causing VEGFR2 hyper-SUMOylation and impaired angiogenic signalling (Fig. 8 . A model for SENP1-mediated VEGFR2 trafficking). Fig. 8 A model for SENP1-mediated VEGFR2 trafficking. SENP1 maintains VEGFR2 in an un-SUMOylated state, ensuring normal trafficking of VEGFR2 from ER/Golgi to plasma membrane in EC. We propose that a pool of VEGFR2 is constantly SUMOylated by an unidentified SUMO E3 ligase in resting EC or upon VEGF-engagement, and stored at the Golgi. Under pathological conditions such as ischemia, SENP1 expression is induced so that SUMOylated VEGFR2 can be rapidly deconjugated and transported to plasma membrane for strong angiogenesis response. Pathological conditions such as hyperglycemia and diabetes downregulate/inactivate SENP1, causing VEGFR2 hyper-SUMOylation and impaired angiogenic signalling as seen in SENP1-deficient EC (see text for details) Full size image Among several post-translational modifications, phosphorylation, ubiquitination, and acetylation of VEGFR2 are well characterized [3] . An early study suggests that the ubiquitin ligase CBL could polyubiquitylate VEGFR2 upon the receptor activation. A later study indicates the F-box-containing E3 ubiquitin ligase βTRCP1, but not CBL, actually ubiquitylates VEGFR2 [13] , [14] , [15] . VEGFR2 ubiquitylation primarily regulates its protein stability and clearance, either through a proteolytic degradation or endocytosis/lysosomal-dependent degradation [13] , [38] . In this regard, ubiquitin-binding protein epsin plays a critical role in VEGF-dependent internalization of VEGFR2 with subsequent targeting to lysosomes for degradation. Our previous study has shown that endothelium-specific deletion of epsin leads to enhanced VEGFR2 signalling and excessive non-productive angiogenesis [12] . Conversely, the de-ubiquitinating enzyme, USP8, is shown to mediate de-ubiquitination of VEGFR2, regulating VEGFR2 trafficking, proteolysis, and signal transduction [39] . Reversible acetylation at lysine residues also regulates VEGFR2 activity [40] . VEGFR2 can be acetylated both at four lysine residues forming a dense cluster in the kinase insert domain and at a single lysine located in the receptor activation loop, and the acetylation significantly alters the kinetics of VEGFR2 phosphorylation after ligand binding by promoting the transition to an open active state, in which tyrosine phosphorylation is favored by better exposure of the kinase target residues [40] , [41] . An important new finding in our study is identification of SUMOylation for VEGFR2. We have performed mass-spectrometry analyses for SUMOylation of VEGFR2 in EC after expression His-tagged SUMO-1. We have detected modifications of Lys1270 by post-translational modifications. However, our mass-spectrometry method cannot distinguish protein SUMOylation and ubiquitylation (W.M., unpublished observations). Further site-specific mutagenesis and co-immunopreciptation assays support the VEGFR2 SUMOylation. Distinct from acetylation, our study indicates that the SUMOylation site lysine1270 is located outside the kinase domain at the very C-terminus of VEGFR2; The alignment attached is a BLAST of the PDB using residues 786–1356 show that the crystal structures all finish at around about residue 1171 (….GNLLQANAQQD 1171 ), which suggests that the C-terminal tail is flexible and more accessible to SUMOylation (as depicted in Figs. 4f and 8 ). SUMOylation may not directly affect the conformation or the kinase activity of VEGFR2, rather prevents its surface targeting and subsequent activation. Results from our current study indicate hyperglycemia induces VEGFR2 SUMOylation, in part, by downregulating SENP1, leading to VEGFR2 accumulation at the Golgi and reduced surface expression. Interestingly, hyperglycemia in mice also increases VEGFR2 ubiquitylation and reduce its expression [36] , [37] . It is important to clearly map the VEGFR2 SUMOylation and ubiquitination under hyperglycemia. A newly identified wild-type α-lytic protease (WaLP, which cleaves peptides after T of the SUMO conjugation …..TGG-K but not after R of the ubiquitin conjugation… RGG-K) and an antibody specific for KGG-peptides have been used to identify specific SUMOylated sites by mass spectrometry [42] . This study provides a useful approach to determine how ubiquitination and SUMOylation coordinately regulate VEGFR2 protein expression and activity under pathological conditions. In addition, the E3 ligase responsible for VEGFR2 SUMOylation has not been identified. Therefore, additional mechanisms for hyperglycemia-induced VEGFR2 SUMOylation need further investigation. The trafficking of newly synthesized VEGFR2 to the plasma membrane is a key determinant of angiogenesis. While VEGFR2 membrane distribution and endocytosis have been extensively investigated [3] . VEGFR2 trafficking to and from other subcellular sites has not been studied. In the present study, we have uncovered a novel mechanism to regulate VEGFR2 cellular trafficking from Golgi to plasma membrane by SUMOylation. Several recent studies have revealed the molecular machinery that carries VEGFR2 from the Golgi to plasma membrane [5] . Syntaxin 6, a Golgi-localised target membrane-soluble N-ethylmaleimide attachment protein receptor (t-SNARE) protein, is shown to mediate VEGFR2 trafficking to the plasma membrane. In another study, the kinesin family plus-end molecular motor KIF13B is shown to deliver VEGFR2 cargo from the Golgi to the EC surface. Specifically, KIF13B is shown to interact directly with VEGFR2 on microtubules [33] . It is plausible that the SUMOylation of VEGFR2 at the terminal domain blocks its association with the exocytotic machinery (e.g., KIF13B) that target VEGFR2 trafficking to plasma membrane, and this hypothesis needs to be further examined. Two reports indicate that VEGFR2 phosphorylation can occur within the Golgi compartment in a VEGF-independent but ROS-dependent manner under hyperglycemia [36] , [37] . The VEGFR2 activation by ROS appears to be non-functional and results in progressively decreased availability of VEGFR2 at the cell surface. These observations promoted us to determine if SENP1-VEGFR2 angiogenic signalling could be impaired by hyperglycemia at diabetic settings. Indeed, hyperglycemia strongly induces downregulation of SENP1 concomitant with VEGFR2 accumulation at the Golgi where it is co-localised with the Golgi marker. VEGFR2 is also accumulated at the Golgi of brain vascular EC isolated from STZ-induced diabetic mice. While STZ mice exhibit reduced VEGF-induced angiogenesis, re-expression of VEGFR2, but not SUMOylated form of VEGFR2, rescues the angiogenesis defects in STZ-induced diabetic mice. Our study supports a critical role of the SENP1-VEGFR2 pathway in the pathological angiogenesis. It has been recognized that certain genes that play important roles in pathological (e.g., inflammation and ischemia) are not involved in physiological angiogenesis. Examples include VEGF homolog placental growth factor (PlGF) [43] and Akt [44] among others. Our own studies show that inflammatory TNFR1 and its associated signalling molecule AIP1, TNF receptor 2 (TNFR2) and its downstream non-receptor tyrosine kinase Bmx are additional members in this group of genes [45] . These studies have led us to postulate that pathological angiogenesis-associated genes are expressed, activated or associated with potent angiogenic pathways in response to pathological stimuli, thereby modulating postnatal angiogenic responses and tissue remodeling. Indeed, we observe an increased SENP1 expression in response to ischemia, correlating the kinetics of VEGFR2-mediated angiogenesis and tissue recovery. Therefore, SENP1 deficiency impairs the VEGFR2 activation and tissue angiogenesis. Conversely, SENP1 is downregulated under pathological conditions such as diabetes, leading to impaired VEGFR2 signalling and angiogenesis. Our study may provide a novel insight into the mechanism by which diabetes impair wound healing in clinic [35] . The exact mechanism for SENP1 upregulation by ischemia and downregulation by hyperglycemia are unknown at present. We observe SENP1 expression in microvessels is induced under ischemia, consistent with the previous finding that induction of SENP1 in EC following exposure to hypoxia. Moreover, the Senp1 gene promoter contains hypoxia response element (HRE) and a mutation on the Senp1 promoter abolishes its transactivation in response to hypoxia [22] . Therefore, the induction of SENP1 in ischemic hindlimb is likely at a transcriptional level driven by HIF1α. Contrasting to hypoxia-induced SENP1 expression, our data indicate that hyperglycemia attenuates SENP1 expression in EC. Hyperglycemia in EC could result in ROS generation [36] , [37] , which is known to modulate SENPs expression and activity [46] , [47] . For example, ROS induce SENP3 thiol modifications and subsequent ubiquitination and degradation. ROS could also modify SENP1 at cysteine residues and attenuate SENP1 activity to increase protein SUMOylation. However, the exact mechanism for SENP1 downregulation by hyperglycemia needs more investigations. Collectively, our in vivo and in vitro studies demonstrate that SENP1 functions as an endogenous activator in VEGFR2 signalling by regulating VEGFR2 trafficking from the Golgi to EC surface. The SENP1-VEGFR2 pathway plays a critical role in pathological angiogenesis in diabetes. Our study suggests that SENP1 may be a novel target for the treatment of diabetes-delayed wound healing. Animals Vascular endothelial cell (EC)-specific deletion of SENP1 (SENP1-ECKO), which was generated by mating SENP1 lox/lox with VE-cadherin-Cre mice [24] , [25] followed by breeding to C57BL/6 background. The deletion of SENP1 in SENP1-ECKO was verified by qRT-PCR using primers amplifying exons 5–6 and specific Cre. SENP1 lox/lox mice were used as controls. We used a standard protocol of STZ injections to induce type I diabetes (T1DM) in C57BL/6 mice. Briefly, C57BL/6 mice at 8 weeks of age mice were injected intraperitoneally with 45 mg/kg STZ or PBS daily for 4 days. Blood glucose concentrations in non-fasting mice were measured 14–16 days after the first injection by an electronic glucometer (Abbott Diabetes Care, Alameda, CA). Blood glucose levels in STZ-treated mice were 350 ± 40 mg/dL (higher than 250 mg/dL were considered diabetic). PBS-treated mice were used as controls for further experiments. Mice were cared for in accordance with National Institutes of Health guidelines, and all procedures were approved by the Yale University Animal Care and Use Committee. In vivo angiogenesis models The study was approved by the Committee of Yale University for Animal Experiments. All experiments were conducted on 8–12 week old male littermates of WT and SENP1-ECKO mice. Mouse hindlimb ischemic model was generated as previously described [28] . Briefly, following anesthesia with combination of 79.5 mg/kg ketamine and 9.1 mg/kg xylazine, the left femoral artery was exposed under a dissecting microscope. The proximal of femoral artery, the distal portion of saphenous artery, and all branches between these two arteries were ligated or cauterized. Then arterectomy was performed. However, for sham operation group, skin incision was done without femoral artery ligation. Blood flow was measured by PeriFlux system with Laser Doppler Perfusion Module (LDPU) unit (Perimed, Inc. North Royalton, OH). Deep measurement probe was placed directly on gastrocnemius muscle to ensure a deep muscle flow measurement. Ischemic and non-ischemic limb perfusion was measured pre-surgery, post-surgery, 3 days, 1 week, 2 weeks and 4 weeks after surgery. The final blood flow values were expressed as the ratio of ischemic to non-ischemic hind limb perfusion. For mouse ear angiogenesis assay, adenovirus encoding VEGF 164 (1 × 10 9 pfu) or same amount of control virus (Ad-LacZ encoding for the β-galactosidase) was intradermally injected into the right and left ear skin of adult mice, respectively. For mouse retina angiogenesis model, Ad-VEGF and Ad-LacZ (1 × 10 8 pfu) were injected into the vitreous humor of right and left eyes, respectively. Five days after viral injection, animal was perfused with PBS and 4% paraformaldehyde (PFA). The ears or retinas were stained with PE-conjugated anti-CD31 to visualize the vascular network. For mouse cornea angiogenesis assay, recombinant human VEGF 165 (generously provided by NIH) was formulated into Hydron pellets at 1 µg/ml and implanted into the cornea of WT and SENP1-ECKO mice as we reported recently [29] . Angiogenesis was assessed by stereomicroscopy on day 5 following implantation, the day of maximum angiogenesis. The contiguous circumferential zone of neovascularization was measured as clock hours using the eye as a 360° circle, and each 30° section as 1 clock hour. Alternatively, vascular area was measured. Animals receiving no treatment were used as positive controls. Implantation of Hydron pellets containing no angiogenic factor was served as negative controls. Fluorescent staining of whole-mount retina, cornea, and ear skin Eyeballs were enucleated and fixed in 4% PFA for 2 h on ice. The cornea, lens, sclera and hyaloid vessels were dissected out and removed [48] . Retinal samples were blocked with 5% normal donkey serum in PBST (0.3%Triton X-100 in PBS) overnight at 4 °C, followed by incubation with isolectin B4 (ThermoFisher Scientific, I21413) diluted 1:50 in blocking solution overnight at 4 °C. After several washes with PBS, retinas were mounted in fluorescent mounting medium. Corneas were carefully dissected out and flattened and postfixed with 4% PFA. The tissues were digested with proteinase K (20 g/mL), followed by whole-mount staining with PE-conjugated anti-CD31 overnight at 4 °C. For ear skin, 20 μl of 1% croton oil (in acetone) was applied on the dorsal side of each ear with a pipette. Mice were sacrificed after 3 h and hair on dorsal side of ear were completely removed with Veet hair remover cream using a cotton swab. Then ears were split into halves and the dorsal ear halves were collected and fixed with acetone at −20 °C for 20 min, followed by whole-mount staining overnight at 4 °C. Images of all samples were obtained using a Leica TCS SP5 confocal microscope (Leica, Germany). Vascular areas analyses were performed using Image J software. Immunofluorescence analysis for tissue sections Mouse muscle and retina tissues were harvested, fixed with 4% PFA and embedded in OCT. [26] 5 μm sections were obtained using a vibratome (Leica). Sections were blocked and permeabilized by overnight incubation in 5% donkey serum and 0.3% TritonX-100 in PBS at 4 °C. Sections were incubated with primary antibodies such as anti-VEGFR2 (1:100) overnight at 4 °C, then were washed with 0.3% TritonX-100 in PBS three times (20 min at 4 °C each) and incubated with secondary antibodies (1:200 to 1:400) at room temperature for 1 h. After secondary antibody incubation, sections were extensively washed twice in 0.3% TritonX-100 in PBS (20 min at 4 °C each) and once in PBS before mounting in VECTASHIELD Mounting medium with DAPI (Vector Laboratory). Micro-CT angiography 2D mCT scans were acquired with a GE eXplore MS Micro-CT System, using a 400 cone-beam with angular increment of 0.5 degrees and 8 to 27 μm slice thickness at a voltage of 163.2 mAs, 80 kVp. mCT data were transferred to a Dell Dimension computer with 3D volume rendering software (version 3.1, Vital Images Inc., Plymouth, MN) and microview software (version 1.15, GE medical system). NIH ImageJ (National Institutes of Health, Bethesda, MD) and Image Pro Plus (Media Cybernatics) software were used to analyze vessel number, diameter, area, volume, and arterial density. Histology and immunohistochemistry Mice were anesthesized and perfused with 10 ml of PBS to wash out the blood throughout the circulatory system. Then tissues were harvested and fixed with 10% buffered formalin. The tissues were embedded in paraffin, sectioned in 5 μM thickness, and sections were stained with routine hematoxylin-eosin or with certain antibodies (e.g., anti-CD31, anti-α-SMA, anti-SENP1, and anti-F4/80) as described previously [28] . Bound primary antibodies were detected using avidin-biotin-peroxidase (NovaRed™ peroxidase substrate kit, Vector Laboratories, Burlingame, CA). All images were taken at least from four areas of each section randomly and sections sections per mice using a light microscope with 40× objective lense. Images were quantified using the Matlab software (The Math Works, Inc. Natick, MA) as described previously [26] . TUNEL assay was performed according to the manufacturer’s instructions (Roche). Gene expression in the tissues Total RNAs were extracted from cultured cells or isolated by mechanical dissociation of fresh dissected tissues using the RNeasy Plus Mini kit (Qiagen) supplemented with β-mercaptoethanol (10 μl/ml). Reverse transcription (RT) into cDNA was achieved according to the manufacturer’s instructions (iScript cDNA Synthesis Kit, Bio-Rad). Quantitative PCR (qPCR) was performed using iQ SYBR Green Master mix on a CFX96 Touch Real-Time PCR Detection System (Bio-Rad). Specific primers (e.g., SENP1, VEGF-A and VEGFR2) were used for qRT-PCR. Isolation of mouse brain endothelial cells Primary mouse brain endothelial cells were isolated by enzymatic digestion from 3-week-old mice. Mice were first anaesthetized and perfused with sterile PBS. Forebrain of the mice were dissected out and meninges were carefully removed away, followed by digestion with 1 mg/ml collagenase type I (Worthington)/dispase (Sigma) in complete DMEM for 1 h at 37 °C with gentle shaking. The digestion was passed through a 100 μm cell strainer (Corning Falcon) Cell pallet was collected by centrifugation (1000 × g , 5 min). Microvessel endothelial cell clusters were separated on a 33% continuous Percoll gradient, and washed twice with DMEM before seeding into collagen type IV and human fibronectin-coated 35-mm plastic dishes. Cultures were maintained in DMEM supplemented with 20% FBS and 1 ng/ml basic fibroblast growth factor (Roche). Upon 90% confluent around day 5, the endothelial cells were passaged with 0.05% trypsin/EDTA solution (Sigma) for further experiments. CD31 + NG2 − MBMVEC and CD31 − NG2 + mouse brain microvessel pericytes (MBMVPC) were isolated from SENP1 lox/lox (WT) and SENP1-ECKO [26] . The expression of SENP1 mRNA and protein were performed by real-time RT-PCR and western blotting, respectively. Cell culture, cytokines, and transfection Human umbilical vein endothelial cell (HUVEC) were from Yale University Vascular Biology and Therapeutics Tissue Culture Core Facility. Human recombinant VEGF (R&D Systems) were used at 10 ng/ml for cell treatment. Plasmid or siRNA transfection of endothelial cells, 293T cells, and COS-7 cells were performed by Lipofectamine 3000 or Lipofectamine RNAiMAX according to Manufacturer’s protocol (Thermo Fisher Scientific), respectively. Around 60–70% confluent, cells were transfected with either plasmid or siRNA. Cells were harvested at 48–72 h post-transfection for indicated experiments. SENP1 siRNAs we used were described previously [49] . CRISPR/Cas9-mediated gene editing for KDR-SUMO1 in human ECs Human endothelial colony forming cell (ECFC)-derived EC were isolated and cultured from umbilical cord blood obtained with informed consent under a protocol approved by the Yale Human Investigation Committee [50] . ECFCs can be passed more times (>15 passages) than HUVECs so they can be used for CRISPR-Cas9-mediated gene editing. We designed a specific single-guide RNA (sgRNA) targeting the vicinity of the stop codon of KDR gene. We also generated the repair template by overlapping PCR containing the 200 bp targeting arms with exon 30 as 5′ arm and 3′UTR of the KDR gene as 3′ arm) flanking the SUMO1 cDNA. The template was digested by lamba exonuclease to prepare single-stranded DNA. Upon CRISPR-Cas9-mediated DNA double-strand breaks were repaired through homologous-directed repair to integrate the SUMO1 cDNA into the KDR locus just before the termination signal [34] (Supplementary Fig. 8 ). This was achieved by nucleofection of cells with pSpCas9(BB)-2A-PuroV2.0 vector that contained expression cassette for the gRNA and a Cas9-2A-Puro along with the single-strand repair template. After 2 days of puro selection, the surviving cells were allowed to grow into colonies. However, the vector was never integrated into the genome, just allowing to be expressed transiently and subsequently degraded. The clones were screened by PCR for modified DNA followed by DNA sequencing. Plasmids and adenovirus Adenoviruses expressing LacZ and VEGF were described previously [29] . Mammalian expression plasmids for VEGFR2 (Flk-1/KDR) and mutants were described previously [51] . Expression plasmids for FLAG-tagged VEGFR2 were generated by inserting human KDR into pcDNA3.FLAG. VEGFR2-WT and mutants were generated by site-mutagenesis using the QuickChange XL-II Site-directed Mutagenesis Kit (Stratagene, La Jolla, CA) as we described previously [51] . Adenovirus-expressing SENP1 and VEGFR2 were generated as we described for AIP1 previously [29] . pAd-SENP1 virus and p-Ad-VEGFR2 were amplified in 293T cells and purified by ultra-centrifugation. Lentiviral expression in EC The Trans-Lentiviral Packaging System was used to express SENP1 and VEGFR2. The plasmids with the coding sequences for SENP1 or VEGFR2 in pLEX MCS vector (Clontech) were transfected and lentiviruses were packed as previously described [26] . MBMVEC or HUVEC were infected with lentivirus supplemented with 8 μg/ml Polybrene (Sigma, St. Louis, MO). Cells were harvested at 36 h post-infection and protein expression was determined by western blot. Immunoprecipitation and immunoblotting Cell lysate preparation, immunoprecipitation and immunoblotting were performed as we previously described [23] . Briefly, cells were washed twice with cold PBS and harvested in a membrane lysis buffer (30 mM Tris, pH 8, 10 mM NaCl, 5 mM EDTA, 10 g/liter polyoxyethylene-8-lauryl ether, 1 mM 0-phenanthroline, 1 mM indoacetamide, 10 mM NaF, 5 mM orthovanadate, 10 mM sodium pyrophosphate). Cell lysates were sonicated and centrifuged at 14,000 × g at 4 °C for 15 min, and supernatants were used immediately for immunoblot or immunoprecipitation. SUMOylation of VEGFR2 was determined by co-immunoprecipitation as we previously described for GATA1 and NEMO proteins [20] , [49] . Antibodies against SENP1, SUMO-1, HIF-1α, phospho-VEGFR2 (pY1054/59), phospho-VEGFR2 (pY1175), phospho-Akt (Ser-473), total VEGFR2 and Akt were from Cell Signalling (Beverly, MA) as described previously [51] . Antibodies against FLAG M2 and HA antibody were from Sigma. Protein A/G PLUS-agarose and anti-β-actin were from Santa Cruz (Santa Cruz, CA). 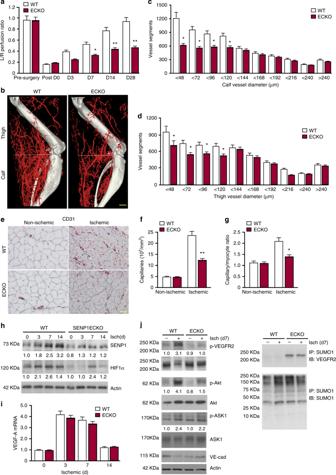Fig. 1 SENP1-ECKO mice exhibit attenuated arteriogenesis and angiogenesis in vivo. WT and SENP1-ECKO mice were subjected to hindlimb ischemic ligation model (HLI).aLaser Doppler analysis of blood flow. The graph shows blood flow in the ischemic foot expressed as a ratio to flow in the normal foot. Quantitative analysis of laser Doppler images indicates significant alterations in hindlimb reperfusion starting at 7 days after femoral artery ligation in SENP1-ECKO mice relative to WT mice (n= 6 each strain).bRepresentative micro-CT images of WT and SENP1-ECKO mice 14 days after HLI.c,dQuantitative micro-CT analysis of arterial vasculature above and below the knee in WT mice (n= 6500 cross-sections per mouse) and SENP1-ECKO mice (n= 4500 cross-sections per mouse) 14 days after common femoral artery ligation. Note a marked decrease in total number of <120-μm-diameter vessels in SENP1-ECKO mice relative to WT littermates in thigh and calf (mean ± SEM, *P< 0.05). Statistical significance was assessed using a Mann–WhitneyUtest and repeated measures analysis performed using one-way nonparametric ANOVA (Kruskal Wallis test).e–gAttenuated angiogenesis in SENP1-ECKO mice. Capillary density was immunostained with an EC marker CD31. Representative sections from non-ischemic and ischemic groups of WT and SENP1-ECKO mice on day 28 post-ischemia are shown in (e). Quantification of capillary density (number/mm2muscle area) and ratio of CD31/myocyte are shown in (f,g). Data are mean ± SEM from ten fields per section (three sections/mouse andn= 4 for each strain).h–jAttenuated VEGF-VEGFR2 signalling in SENP1-ECKO. Muscle tissues from WT and SENP1-ECKO were harvested at various days post-ischemia as indicated.hHIF-1α, SENP1, and β-actin were determined by western blot with respective antibodies.iVEGF-A mRNA was measured by qRT-PCR with GAPDH for normalization. Fold changes are presented.n= 2 per group.jPhosphorylations of VEGFR2, Akt, and ASK1 as well as total proteins as indicated in tissue lysates were determined by western blot with respective antibodies. SUMOylated VEGFR2 was determined by co-immunoprecipitation assays with anti-SUMO1 followed by western blotting with anti-VEGFR2. Protein bands in (h,j) were quantified by densitometry and fold changes are presented by taking WT non-ischemia as 1.0.n= 2. Error bars, mean ± SEM;∗P< 0.05, **P< 0.01, one-way ANOVA. Scale bar: 500 μm (b); 20 μm (e) All antibodies used are listed in Supplementary Table 1 . 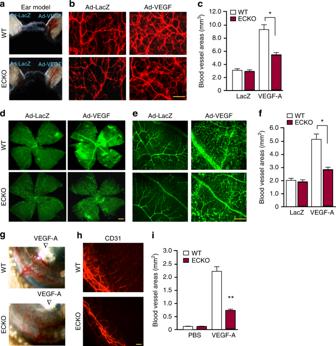Fig. 2 VEGF-induced retina and cornea neovascularization were greatly attenuated in SENP1-ECKO mice.a–cVEGF-induced ear angiogenesis. Adenovirus encoding VEGF164(1 × 109pfu) (Ad-VEGF) or β-galactosidase (Ad-LacZ) was intradermally injected into the mice right and left ear skin, respectively.aVEGF-induced angiogenesis in WT and SENP1-ECKO mice was accessed by a direct microscopy.bEar vasculature was visualized by a whole-mount staining with PE-conjugated anti-CD31.cQuantification of vessel density from 10 fields per ear (n= 5 for each group).d–fVEGF-induced retina angiogenesis. Ad-VEGF or Ad-LacZ (1 × 109pfu) was injected intravitreously into WT and SENP1-ECKO mice. Retina vasculature was visualized by isolectin staining (low power images in (d) and high power images in (e) with quantification of vessel density in (f).g–iVEGF-induced cornea angiogenesis assay. A Hydron pellet containing VEGF protein was implanted into the cornea of WT and SENP1-ECKO mice. Angiogenesis was assessed by stereomicroscopy on day 5 following implantation (g) and immunostaining with anti-CD31 (h). Vascular density was quantified in (i). Quantificaitons were from ten fields per tissue (ear, retina or cornea) (n= 5 for each group). Error bars, mean ± SEM;∗P< 0.05, **P< 0.01, one-way ANOVA. Scale bar: 100 μm (b,e,h); 400 μm (d) Uncropped scans of the original western blots are shown in Supplementary Fig. 10 – 11 . Biotinylation of cell surface VEGFR2 VEGFR2 surface expression was measured as described previously [12] . MBMVEC were starved overnight before being treated with 50 ng/ml of VEGF-A for 0, 5, 15 or 30 min at 37 °C to allow internalization of cell surface VEGFR2. At the end point of treatment, cells were incubated with 1 mM EZ-Link Sulfo-NHS-LC-Biotin on ice for 30 min, washed with 50 mM glycine followed by cell lysis with RIPA buffer and processed for streptavidin bead pull down. Cell surface biotinylated VEGFR2 was visualized by western blotting using anti-VEGFR2 antibodies and quantified by NIH Image J software. Monolayer endothelial cell migration assay This assay was modified as described previously [51] . Transfected monolayer endothelial cells were cultured in 0.5% FBS for serum starvation and then subjected to “wound injury” with a 200 μl pipette tip. After changing with fresh media, cells were further cultured for 12–24 h. “Wound” areas were measured to evaluate EC migration. Images were captured under a Zeiss Axiovert microscope (10×). EC tube formation assay Fifty-microliters of Matrigel was evenly distributed to each well of 96-well plates, and incubated for 30 min at 37 °C (Matrigel, Becton Dickinson, Bedford, MA). Cells at early passages (e.g., P2-P5) were re-suspended with serum-free media. Add 100 μl (1–2 × 10 4 ) of single cell suspension on top of Matrigel to each well. After 30 min, fresh media with 10 ng/ml of VEGF was added and further incubated at 37 °C for 4–24 h. Each conditional group contained four wells. Tubules network in each well were imaged from 3 to 5 random fields using a Leica (Bannockbern, IL) phase contrast microscope and analyzed by NIH Image 1.60. Three-dimensional bead sprouting assay Control or SENP1 siRNA was transfected into HUVECs for 8 h by Lipofectamine RNAiMAX according to the manufacturer’s protocol (Invitrogen). Carefully removed the media from the cells and added fresh Microvascular Endothelial Cell Growth Medium-2 MV (EGM2, Lonza) into transfected cells. WT human EC and KDR-SUMO1 knockin EC were cultured in normal EGM2 media. Based on a published protocol [52] , three-dimensional bead sprouting assay was performed. Twenty-four hours post-transfection, cells were trypsinized and centrifuged with 1000 rpm for 5 min. Cell pellets were coated with Cytodex 3 microcarrier beads (C3275, Sigma) in EGM2 medium in a condition of 400 cells per bead. To make fibrin gels, 2 mg/ml fibrinogen (Calbiochem) in DPBS, 0.625 U/mL thrombin (Sigma-Aldrich), and 0.15 Units/ml aprotinin (Sigma-Aldrich) were mixed. Immediately, coated beads were embedded into fibrin gels, and 500 μl of suspension were seeded slowly to each well in 24-well plates. A total of 20,000 fibroblasts in 1 ml EGM2 medium was added on top of fibrin gels in each well. The cells were cultured and maintained for 2–8 days by changing the medium every other day. 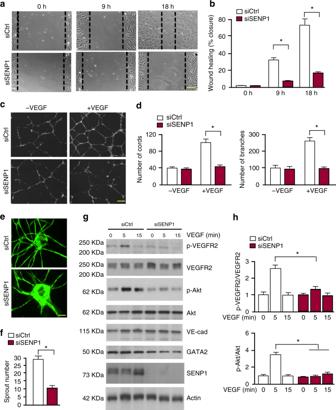Fig. 3 VEGF-induced angiogenic responses were inhibited by SENP1 silencing. HUVEC were transfected with control siRNA (siCtrl) or SENP1 siRNA (siSENP1) for 24 h. Cells were cultured in 0.5% FBS for overnight and subjected to EC migration and tube formation in response to VEGF (10 ng/ml).a,bEC migration by a scratch assay for indicated times. Wound healing (% closure) was quantified.c,dEC tube formation in a Matrigel assay. Representative images are shown in (c). Number of cords and branches were quantified from ten fields per group (d).e,f3D spheroid sprouting assay. siRNA-transfected HUVECs were infected with EGFP-expressing retroviruses. Cells were coated with microbeads, embedded in fibrin gels and grown in EGM2 medium for 8 days.eA representative image of ten beads for each sample is shown.fQuantification of sprout number is shown in panel. Three independent experiments were performed.g,hCtrl siRNA and SENP1 siRNA HUVEC were cultured overnight in 0.5% FBS followed by VEGF treatment (10 ng/ml) for indicated times (0–15 min).gPhosphorylation of VEGFR2 and Akt as well as the total proteins as indicated were determined by western blot with respective antibodies.hProtein bands were quantified by densitometry and fold changes are presented by taking untreated siCtrl group as 1.0.n= 2. Error bars, mean ± SEM;∗P< 0.05, Studentt-test (f) or one-way ANOVA. Scale bar: 1 mm (a,c,e) Bright field images were took under Axiovert 200 (Zeiss) microscope at 10× magnification and sprout lengths were measured by NIH Image J. Immunofluorescence microscopy (IF) Cells were grown on fibronectin-coated glass chamber slides (VWR Scientific International), fixed with 4% PFA in PBS for 15 min at room temperature, permeabilised with 0.1% triton-X buffer, blocked in 5% donkey serum diluted in PBS for 1 h and stained 2 h at room temperature or 4 °C overnight using specified antibodies, followed by Alexa Fluor 488- or 594-conjugated secondary antibodies (Invitrogen Molecular Probes, Eugene, OR). Slides were observed using a Zeiss Axiovert 200 fluorescence microscope (Carl Zeiss MicroImaging; Thornwood, NY), and images were captured using Openlab3 software (Improvision, Lexington, MA). Study design and statistical analysis Animal were grouped with no blinding but randomized during the experiments. Male and female animals were used in equal numbers for all experiments. No samples or animals were excluded from analysis. Group sizes were determined by an a priori power analysis for a two-tailed, two-sample t -test with an α of 0.05 and power of 0.8, in order to detect a 10% difference at the endpoint. All quantifications (clinical score, hindlimb flow, in vivo and in vitro angiogenesis, VEGFR2 cellular localisations) were performed in a blind fashion. All figures are representative of at least two experiments unless otherwise noted. All graphs report mean ± SEM values of biological replicates. Comparisons between two groups were performed by unpaired, two-tailed t -test, between more than two groups by one-way ANOVA followed by Bonferroni’s post hoc or by two-way ANOVA using Prism 6.0 software (GraphPad). P values were two-tailed and values <0.05 were considered to indicate statistical significance. P < 0.05, P < 0.01, and P < 0.001 are designated in all figures with *, **, ***, respectively. 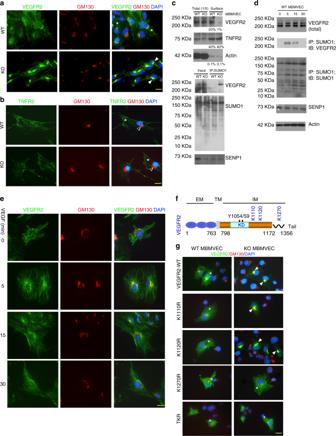Fig. 4 SUMOylation of VEGFR2 at the C-terminal lysine-1270 retains VEGFR2 in the Golgi.a,b. MBMVEC isolated from WT and SENP1-ECKO mice were subjected to immunofluorescence staining for VEGFR2 (a) or TNFR2 (b) together with a Golgi marker GM130.cWT and SENP1-ECKO MBMVECs were cultured in normal media. Cell-surface VEGFR2 was labeled by cell-surface biotinylation, and analyzed by streptavidin bead pull-down followed by western blotting with anti-VEGFR2. Percentage of cell-surface vs total proteins (VEGFR2, TNFR2 and actin) were quantified.n= 2.dCell lysates of MBMVEC isolated from WT and SENP1-ECKO mice were subjected to western blot for total SENP1, VEGFR2, and co-immunoprecipitation assays for VEGFR2 SUMOylation. Relative molecular weights are shown on the left.eWT MBMVEC were treated with VEGF (10 ng/ml) for indicated times, and cells were subjected to immunofluorescence staining for co-localisation of VEGFR2 with GM130 (e).fSchematic diagram of VEGFR2 domains. EM: extracellular domain, TM: transmembrane domain, IM: intracellular domain, Tail: a flexible C-terminal segment (residues aa1172–1356). The numbers refer to the amino acid number, indicating the boundary of each domain. Y1054/59 located at the activation loop and putative SUMO sites within the IM (K1110, K1120, and K1270) are indicated. All VEGFR2 expression constructs are Flag-tagged at the N termini.gVEGFR2-WT and mutants were transfected into WT or SENP1-deficient MBMVEC. Co-localisation of VEGFR2 (anti-FLAG) with GM130 was determined. Merged images are shown (see Supplementary Fig.6for split channel images). A total of 10 cells from each group were analyzed. Golgi-accumulated VEGFR2 is indicated by arrows while membrane/cytosolic VEGFR2 by asterisks (a,b,e,g). TNFR2 was absent in Golgi (b). Three independent experiments were performed. Scale bar, 20 μm (a,b,e,g) 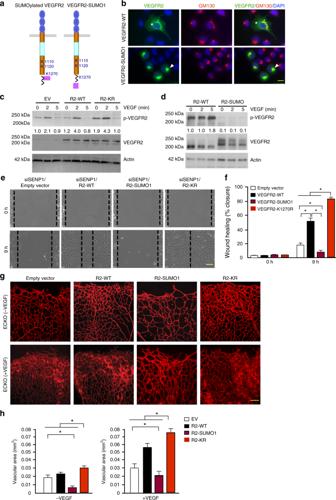Fig. 5 SUMOylation of VEGFR2 blocks VEGFR2 surface targeting and VEGFR2-mediated angiogenesis.aSchematic diagram of VEGFR2-SUMO1 fusion compared to endogenous SUMOylated VEGFR2.bHUVECs were transfected with VEGFR2-WT or VEGFR2-SUMO1, and cells were co-immunostained with anti-VEGFR2 and GM130. Merged images with DAPI counterstaining (blue) are shown. A total of 10 cells from each group were analyzed. Golgi-accumulated VEGFR2 is indicated by arrows while membrane/cytosolic VEGFR2 by asterisks.c,dHUVECs were infected with lentivirus expressing empty vector (EV), VEGFR2-WT, VEGFR2-KR or VEGFR2-SUMO1 followed by VEGF treatment as indicated. Phosphor- and total VEGFR2 were examined by western blotting. Protein bands were quantified by densitometry and fold changes are presented by taking untreated VEGFR2-WT group as 1.0.n= 2.e,fHUVEC were infected with lentivirus expressing empty vector, VEGFR2-WT, VEGFR2-SUMO1 and VEGFR2-K1270R for 24 h. Cells were cultured in 0.5% FBS for overnight and subjected to EC migration in response to VEGF (10 ng/ml). Representative images are presented in (e) and wound healing (% closure) at 9 h was quantified in (f). Data are mean ± SEM from ten fields per group. Three independent experiments were performed.g,hVEGFR2-SUMO1 blunts retina angiogenesis. Ad-VEGF or Ad-LacZ (1 × 109pfu) was co-injected intravetrously with VEGFR2-WT, VEGFR2-SUMO1 or VEGFR2-K1270R into 4 day-old pups. Retina was harvested on day 5 post-injection and retina vasculature was visualized by isolectin staining with confocal images in (g) with quantification of vessel density in (h).n= 5 for each group. Error bars, mean ± SEM;∗P< 0.05, one-way ANOVA. Scale bar, 20 μm (b); 1 mm (e); 100 μm (g) 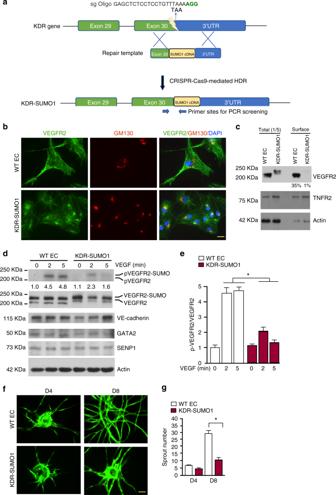Fig. 6 VEGFR2-SUMO1 fusion in human EC inhibits VEGF-mediated angiogenesis.aSchematic diagram of KDR-SUMO1 knockin in human EC by CRISPR/Cas9-mediated gene editing. A specific sgRNA targeting the vicinity of the stop codon of KDR gene encoding VEGFR2 and a repair template containing targeting arms with exon 30 as 5′ arm and the 3′UTR of the KDR gene as 3′ arm flanking the SUMO1 cDNA. Upon CRISPR/Cas9-mediated DNA double-strand breaks were repaired through homologous-directed repair, the SUMO1 cDNA was integrated into the KDR locus just before the termination signal. The PCR primers used for screening for KDR-SUMO1 fusion clones are indicated.bWT human EC and KDR-SUMO1 knockin EC were subjected to immunofluorescence staining for co-localisation of VEGFR2 with GM130. Similar pattern localisation was observed in cells derived from additional two clones.cWT human EC and KDR-SUMO1 knockin EC were cultured in normal media. Cell-surface VEGFR2 was labeled by cell-surface biotinylation, and analyzed by streptavidin bead pull-down followed by western blotting with anti-VEGFR2. Percentage of cell-surface VEGFR2 vs total VEGFR2 in WT EC and KDR-SUMO1 EC were quantified.n= 3.d,eWT human EC and KDR-SUMO1 knockin EC were treated with VEGF (10 ng/ml) for indicated times, and cells were subjected to western blot for VEGFR2 phosphorylation (c). Protein bands were quantified by densitometry and fold changes are presented by taking untreated WT group as 1.0 (d).n= 2.f,g3D spheroid sprouting assay. Human ECs were infected with EGFP-expressing retroviruses. Cells were coated with microbeads, embedded in fibrin gels and grown in EGM2 medium for 8 days. A representative image of ten beads for each sample is shown (f). Quantification of sprout number is shown in panel (g). Three independent experiments were performed. Error bars, mean ± SEM; *P< 0.05, one-way ANOVA. Scale bar: 20 μm (b); 1 mm (f) 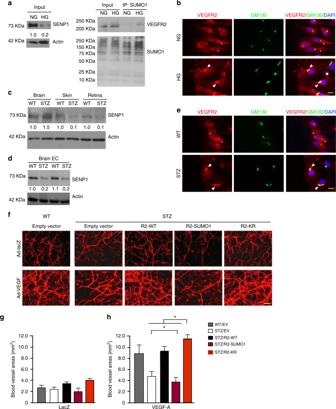Fig. 7 The SENP1-VEGFR2 signalling in diabetic angiogenesis.a,bHUVEC were cultured under 5 mM or 25 mM glucose for 72 h. Expression of SENP1 and VEGFR2 SUMOylation were determined (a). VEGFR2 localisation was determined by indirect immunofluorescence for VEGFR2 and GM130 (b).cTissues from WT and STZ mice were harvested. SENP1 expression in brain (whole lysates), retina and ear skin (the vascular layer) was determined by western blot with anti-SENP1.dSENP1 expression in MBMVEC isolated from WT and STZ mice. Protein bands in (c,d) were quantified by densitometry and fold changes are presented by taking WT group as 1.0.n= 2.eVEGFR2 localisation in MBMVEC isolated from WT and STZ mice was determined by indirect immunofluorescence for VEGFR2 and GM130.f–hAdenovirus encoding VEGF164(1 × 109pfu) (Ad-VEGF) or β-galactosidase (Ad-LacZ) was co-injected with empty vector, VEGFR2-WT, VEGFR2-SUMO1 or VEGFR2-K1270R intradermally into ear skin of SENP1-ECKO mice. VEGF-induced angiogenesis in WT and SENP1-ECKO mice was accessed by a whole-mount staining with anti-CD31 antibody. Vascular density was quantified and data are mean ± SEM from ten fields per mouse ear. (n= 5 for each group). Error bars, mean ± SEM; *P< 0.05, one-way ANOVA. Scale bar: 20 μm (b); 100 μm (f) 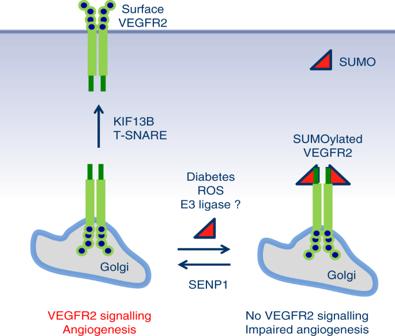Fig. 8 A model for SENP1-mediated VEGFR2 trafficking. SENP1 maintains VEGFR2 in an un-SUMOylated state, ensuring normal trafficking of VEGFR2 from ER/Golgi to plasma membrane in EC. We propose that a pool of VEGFR2 is constantly SUMOylated by an unidentified SUMO E3 ligase in resting EC or upon VEGF-engagement, and stored at the Golgi. Under pathological conditions such as ischemia, SENP1 expression is induced so that SUMOylated VEGFR2 can be rapidly deconjugated and transported to plasma membrane for strong angiogenesis response. Pathological conditions such as hyperglycemia and diabetes downregulate/inactivate SENP1, causing VEGFR2 hyper-SUMOylation and impaired angiogenic signalling as seen in SENP1-deficient EC (see text for details) Data availability All other data supporting the presented findings are available from the corresponding author upon request.